Toll-like receptor 3 recognizes incomplete stem structures in single-stranded viral RNA Endosomal Toll-like receptor 3 (TLR3) serves as a sensor of viral infection and sterile tissue necrosis. Although TLR3 recognizes double-stranded RNA, little is known about structural features of virus- or host-derived RNAs that activate TLR3 in infection/inflammatory states. Here we demonstrate that poliovirus-derived single-stranded RNA segments harbouring stem structures with bulge/internal loops are potent TLR3 agonists. Functional poliovirus-RNAs are resistant to degradation and efficiently induce interferon-α/β and proinflammatory cytokines in human and mouse cells in a TLR3-dependent manner. The N- and C-terminal double-stranded RNA-binding sites of TLR3 are required for poliovirus-RNA-mediated TLR3 activation. Like polyriboinosinic:polyribocytidylic acid, a synthetic double-stranded RNA, these RNAs are internalized into cells via raftlin-mediated endocytosis and colocalized with TLR3. Raftlin-associated RNA uptake machinery and the TLR3 RNA-sensing system appear to recognize an appropriate topology of multiple RNA duplexes in poliovirus-RNAs. Hence, TLR3 is a sensor of extracellular viral/host RNA with stable stem structures derived from infection or inflammation-damaged cells. Type I interferon (IFN) production is crucial for controlling virus infections [1] , [2] . Toll-like receptors (TLRs) 3, 7, 8 and 9 and RIG-I-like receptors detect viral nucleic acids in the endosomes and cytoplasm, respectively, and induce cytokine production, including type I IFNs (IFN-α and IFN-β), via distinct adaptor proteins [3] . TLR3 recognizes double-stranded RNA (dsRNA), a viral replication intermediate that is produced by positive-strand RNA viruses and DNA viruses, and signals to produce IFN-β and proinflammatory cytokines through the Toll-interleukin-1 (IL-1) receptor domain-containing adaptor molecule-1 (TICAM-1, also known as TRIF) [4] , [5] , [6] , [7] , [8] . TLR3 is expressed at high levels in myeloid dendritic cells (DCs), especially in professional antigen-presenting DCs, such as mouse splenic CD8α + DCs and human CD141 + DCs, and localizes to the early endosome [9] , [10] , [11] . Although macrophages, fibroblasts and epithelial cells also express TLR3 on the cell surface as well as the endosomal membrane, TLR3-mediated signalling initiates from the endosomal compartment [12] . Thus, TLR3 activation depends on the uptake of extracellular virus-derived RNA molecules. Studies using TLR3-deficient mice demonstrated that TLR3 mediates a protective response against positive-strand RNA virus infection, including coxsackie virus group B serotype 3, encephalomyocarditis virus and poliovirus (PV), all of which belong to the Picornaviridae family [13] , [14] , [15] , [16] . TLR3- or TICAM-1-deficient human PV receptor (PVR)-transgenic mice were more susceptible than normal PVR-transgenic mice to intraperitoneal or intravenous inoculation with a low titre of PV [15] , [16] . TLR3-dependent type I IFN production by splenic CD11c + DCs and macrophages was essential for the protection of PVR-transgenic mice against PV infection. In addition to mouse studies, genetic studies in the patients with herpes simplex encephalitis demonstrated that the TLR3-TICAM-1 pathway is involved in the protection against herpes simplex virus-1 encephalitis in children [17] , [18] , [19] . Collectively, these findings indicate that TLR3 has an important role in anti-viral responses in both humans and mice. However, several studies have also demonstrated that TLR3-mediated signalling exacerbates RNA virus infection including West Nile virus (positive-strand RNA virus), influenza virus and phelebovirus (negative-strand RNA viruses) [20] , [21] , [22] . TLR3-dependent inflammatory cytokine and chemokine productions have an impact on virus-induced pathology and host survival, and, remarkably, RNA from necrotic cells or host mRNA are also recognized by TLR3 [23] , [24] . However, RNA species detected by TLR3 have not been analysed and little is known about the essential structural elements of virus- or host-derived RNAs capable of activating TLR3 in an infection/inflammatory state. In the current study, we analysed the RNA structure recognized by TLR3 using in vitro -transcribed RNAs derived from PV. We found that, in addition to dsRNA, PV-derived structured RNAs harbouring ds regions with bulges and internal loops are potent TLR3 ligands. The PV-RNAs activated endosomal TLR3 in mouse and human cells, leading to the production of IFN-α/β and proinflammatory cytokines. Identification of RNA structures recognized by TLR3 To examine whether viral RNA activates TLR3 extracellularly, mouse splenic DCs from wild-type (WT) or TLR3-deficient mice were stimulated with total RNA isolated from PV-infected or uninfected Vero cells, or a synthetic viral dsRNA analogue, polyriboinosinic:polyribocytidylic acid (poly(I:C)), in FCS-free medium. Poly(I:C) induced type I IFN production by mouse splenic DCs in a TLR3-independent manner ( Fig. 1a ). The results reflect a current notion that cytosolic RNA helicase, melanoma differentiation-associated gene 5 (MDA5), in addition to endosomal TLR3, senses poly(I:C) to induce type I IFNs in mouse DCs [25] . However, this is not the case in RNA from PV-infected cells, which induces type I IFNs and proinflammatory cytokines in splenic DCs largely through their TLR3 ( Fig. 1a and Supplementary Fig. S1 ). Notably, RNA from PV-uninfected cells had no potential for IFN/cytokine induction ( Fig. 1a and Supplementary Fig. S1 ). Given that PV infection leads to a rapid inhibition of host-cell RNA synthesis [26] , the main RNA species in PV-infected Vero cells were approximately 8,000-nucleotide (nt) RNA corresponding to the PV genome and its replicative form, which were segmented into approximately 1,000–2,000-nt RNAs in the FCS-free culture medium ( Fig. 1b ). The ~8,000-nt PV-RNAs were degraded by treatment with single-stranded RNA (ssRNA)- and dsRNA-specific RNase, suggesting the existence of ss and ds forms of PV-derived RNAs in PV-infected cells ( Supplementary Fig. S2 ). 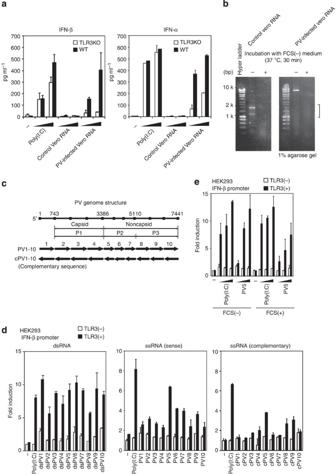Figure 1: Extracellular PV-RNAs induce TLR3-mediated type I IFN production. (a) Mouse splenic CD11c+DCs from WT or TLR3−/−mice (1 × 106per ml) were stimulated with medium alone (−), poly(I:C), total RNA from PV-infected Vero cells or total RNA from uninfected Vero cells (25, 100 μg ml−1) for 24 h in FCS(−) AIM-V medium. RNAs were pre-treated with polymyxin B (5 μg ml−1) for 1 h before addition. IFN-α/β levels in culture supernatants were measured using ELISA. Representative data from three independent experiments are shown (mean±s.d.). (b) The RNA extracted from PV-infected or uninfected Vero cells was incubated in FCS(−) AIM-V medium for 30 min and then electrophoresed on a 1% agarose gel. The PV-RNAs were segmented into approximately 1,000–2,000-nt RNAs in FCS-free medium (right panel, square bracket). (c) Constructs ofin vitro-transcribed PV-RNAs. Diagram of PV genome is shown (Top). Coding regions for viral capsid proteins (P1) and noncapsid proteins (P2 and P3) are indicated. Positions of the sense RNAs (PV1–10) and the complementary RNAs (cPV1–10) corresponding to the PV genome are shown as arrows. Each starting and ending position and length are described inSupplementary Table S1. (d) PV-RNA-induced TLR3-mediated IFN-β promoter activation. HEK293 cells were transfected with an empty vector (−) or expression plasmid for TLR3, together with the IFN-β promoter reporter and phRL-TK. Twenty-four hours after transfection, culture media was removed and 10 μg ml−1poly(I:C), PV-derived dsRNAs, dsPV1–dsPV10 (left panel), sense RNAs, PV1–PV10 (middle panel) or complementary RNAs, cPV1–cPV10 (right panel), were added with FCS-free medium. Luciferase activity was measured 6 h after stimulation and shown as mean fold index induction compared with non-stimulated cells. Representative data from three independent experiments are shown (mean±s.d.). (e) Effect of FCS on the PV5-induced TLR3-mediated IFN-β promoter activation. Cells were stimulated with increasing amounts of poly(I:C) or PV5 (2.5, 10 or 25 μg ml−1) in the condition of FCS-free or -containing medium. Figure 1: Extracellular PV-RNAs induce TLR3-mediated type I IFN production. ( a ) Mouse splenic CD11c + DCs from WT or TLR3 −/− mice (1 × 10 6 per ml) were stimulated with medium alone (−), poly(I:C), total RNA from PV-infected Vero cells or total RNA from uninfected Vero cells (25, 100 μg ml −1 ) for 24 h in FCS(−) AIM-V medium. RNAs were pre-treated with polymyxin B (5 μg ml −1 ) for 1 h before addition. IFN-α/β levels in culture supernatants were measured using ELISA. Representative data from three independent experiments are shown (mean±s.d.). ( b ) The RNA extracted from PV-infected or uninfected Vero cells was incubated in FCS(−) AIM-V medium for 30 min and then electrophoresed on a 1% agarose gel. The PV-RNAs were segmented into approximately 1,000–2,000-nt RNAs in FCS-free medium (right panel, square bracket). ( c ) Constructs of in vitro -transcribed PV-RNAs. Diagram of PV genome is shown (Top). Coding regions for viral capsid proteins (P1) and noncapsid proteins (P2 and P3) are indicated. Positions of the sense RNAs (PV1–10) and the complementary RNAs (cPV1–10) corresponding to the PV genome are shown as arrows. Each starting and ending position and length are described in Supplementary Table S1 . ( d ) PV-RNA-induced TLR3-mediated IFN-β promoter activation. HEK293 cells were transfected with an empty vector (−) or expression plasmid for TLR3, together with the IFN-β promoter reporter and phRL-TK. Twenty-four hours after transfection, culture media was removed and 10 μg ml −1 poly(I:C), PV-derived dsRNAs, dsPV1–dsPV10 (left panel), sense RNAs, PV1–PV10 (middle panel) or complementary RNAs, cPV1–cPV10 (right panel), were added with FCS-free medium. Luciferase activity was measured 6 h after stimulation and shown as mean fold index induction compared with non-stimulated cells. Representative data from three independent experiments are shown (mean±s.d.). ( e ) Effect of FCS on the PV5-induced TLR3-mediated IFN-β promoter activation. Cells were stimulated with increasing amounts of poly(I:C) or PV5 (2.5, 10 or 25 μg ml −1 ) in the condition of FCS-free or -containing medium. Full size image A functional screening for PV-derived ssRNA and dsRNA was performed using an IFN-β promoter reporter assay to determine the RNA structure recognized by TLR3. Approximately 540–920 nts contiguous sense (PV1–10) or complementary (cPV1–10) RNAs and their dsRNA forms (dsPV1–10) were transcribed in vitro using PV-cDNA as a template ( Fig. 1c and Supplementary Table S1 ), and their TLR3-activating ability was assessed. HEK293 cells transfected with the TLR3-expression vector or empty vector, together with the IFN-β promoter reporter plasmid, were stimulated with PV-RNAs in FCS-free or FCS-containing media. All PV-derived dsRNAs induced TLR3-dependent IFN-β promoter activation similar to poly(I:C) ( Fig. 1d , left panel). Interestingly, several PV-ssRNAs, either sense or complementary RNA, also activated the IFN-β promoter through TLR3 in FCS-free medium ( Fig. 1d , centre and right panels). We further examined the effect of FCS on the IFN-β-inducing abilities of PV-RNAs using PV5. PV5 retained TLR3-activating ability, even in the FCS-containing medium ( Fig. 1e ). To explore the relationship between TLR3-activating capacity and the degradability of PV-RNAs, PV-RNAs were incubated in FCS(−) or FCS(+) medium for 30 min at 37 °C and then subjected to agarose gel electrophoresis. Non-functional PV-RNAs were readily degraded in the FCS(−) or FCS(+) medium, whereas functional RNAs, including high-potential PV5 and cPV5 and low-potential PV6, were stable before and after incubation in the FCS(+) medium ( Fig. 2a ). Correspondingly, dose-dependent TLR3 activation was observed with PV5 and PV6 but not with others including cPV1 ( Fig. 2b ). Notably, these PV-RNAs stimulated the cytosolic RNA sensors when transfected into cells ( Supplementary Fig. S3a ). TLR3-mediated IFN-β promoter activation was also observed with PV5- or cPV5-containing long-size PV-RNAs, although the activity was less than that of PV5 ( Supplementary Fig. S3b and Supplementary Table S1 ). In addition, segmentation of PV5 into three ~200-nt RNAs (PV5 a, b and c) destroyed the activity of intact PV5, despite the fact that these RNA segments were resistant to degradation ( Supplementary Fig. S3c and Supplementary Table S1 ). These results suggested that an appropriate length of PV-RNAs with a stable structure activate endosomal TLR3, inducing IFN-β promoter activation. 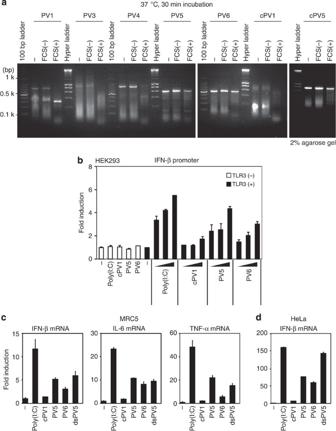Figure 2: PV-ssRNA-induced TLR3 activation is correlated with the degradability of RNAs. (a) PV-RNAs were incubated in cell-free FCS-free or -containing medium at 37 °C. Non-treated RNA or RNA incubated for 30 min were loaded onto a 2% agarose gel. (b) HEK293 cells transiently expressing TLR3 were stimulated with increasing amounts of poly(I:C), cPV1, PV5 or PV6 (2.5, 10 or 25 μg ml−1) for 6 h. HEK293 cells transfected with empty vector were stimulated with 25 μg ml−1poly(I:C) or indicated PV-RNA. IFN-β promoter activation is shown as mean fold index induction compared with non-stimulated cells. Representative data from three independent experiments are shown. (c,d) IFN-β mRNA expression induced by PV-RNAs in human cells expressing TLR3. MRC5 cells (c) or HeLa cells (d) in FCS(−) AIM-V medium were stimulated with 20 μg ml−1poly(I:C) or PV-derived RNAs for 3 h. Total RNA was extracted and quantitative PCR was performed using primers for the respective genes. Expression of each gene was normalized to glyceraldehyde 3-phosphate dehydrogenase mRNA expression. Data are shown as the mean±s.d. Representative data from three independent experiments are shown. Figure 2: PV-ssRNA-induced TLR3 activation is correlated with the degradability of RNAs. ( a ) PV-RNAs were incubated in cell-free FCS-free or -containing medium at 37 °C. Non-treated RNA or RNA incubated for 30 min were loaded onto a 2% agarose gel. ( b ) HEK293 cells transiently expressing TLR3 were stimulated with increasing amounts of poly(I:C), cPV1, PV5 or PV6 (2.5, 10 or 25 μg ml −1 ) for 6 h. HEK293 cells transfected with empty vector were stimulated with 25 μg ml −1 poly(I:C) or indicated PV-RNA. IFN-β promoter activation is shown as mean fold index induction compared with non-stimulated cells. Representative data from three independent experiments are shown. ( c , d ) IFN-β mRNA expression induced by PV-RNAs in human cells expressing TLR3. MRC5 cells ( c ) or HeLa cells ( d ) in FCS(−) AIM-V medium were stimulated with 20 μg ml −1 poly(I:C) or PV-derived RNAs for 3 h. Total RNA was extracted and quantitative PCR was performed using primers for the respective genes. Expression of each gene was normalized to glyceraldehyde 3-phosphate dehydrogenase mRNA expression. Data are shown as the mean±s.d. Representative data from three independent experiments are shown. Full size image PV-RNAs induce IFN-β production by human fibroblasts We next examined whether PV-RNAs induced IFN-β production from human fibroblasts and epithelial cells that endogenously expressed TLR3. MRC5 cells were stimulated with cPV1, PV5, PV6 or dsPV5 extracellulary, and IFN-β mRNA was assessed using quantitative PCR (qPCR). PV5 and PV6 induced IFN-β mRNA expression in MRC5 cells similar to dsPV5 stimulation ( Fig. 2c ). mRNA encoding the proinflammatory cytokines, IL-6 and TNF-α, were also induced by PV5, PV6 or dsPV5. Similarly, HeLa cells greatly increased IFN-β mRNA expression in response to PV5, PV6 or dsPV5 ( Fig. 2d ). In contrast, cPV1 did not induce any cytokine mRNA transcription from MRC5 and HeLa cells. TLR3 recognizes PV-RNA through the dsRNA-binding sites Biochemical studies using in vitro -transcribed dsRNAs have shown that relatively long stretches of dsRNA (>90 bp in length) are required for TLR3-mediated IFN-β promoter activation in HEK293/TLR3 cells and cytokine production from mouse myeloid DCs [11] , [27] . To determine the structural features of TLR3-activating or non-activating RNAs, the secondary structure of PV-RNAs was predicted using the mfold WebServer program, which calculates the minimum free-energy secondary structure [28] . Each PV-RNA contains ds (<11 bp in length) and ss regions, and, intriguingly, the percentages of stem/loop structure were almost the same in each PV-RNA ( Fig. 3a ). However, the secondary structure models of cPV1, PV5 and PV6 have clearly showed that cPV1 contains multiple branched stems and large loop structures that may be targeted by RNases, whereas functional PV5 and PV6 possess tandemly arranged ds regions, which were segmented with bulge or internal loops. Thus, RNAs that we prepared are not a typical ds structure of the TLR3 ligand. The topology of multiple dsRNA regions and the overall secondary and tertiary structures of PV-RNAs appear to influence the stability and TLR3-activating ability. 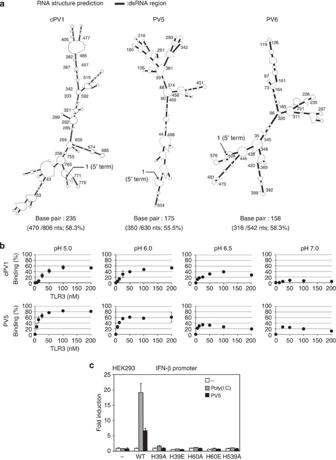Figure 3: Both N- and C-terminal dsRNA-binding sites of TLR3 are required for PV-RNA-induced TLR3 activation. (a) Secondary structure of PV-RNAs (cPV1, PV5 and PV6) predicted by the mfold software. Thick lines indicate dsRNA regions (1–11 bp). The starting and ending positions of ds regions are shown with the nt number. A total number of base pair and the number of nts involved in base pairing in cPV1, PV5 and PV6 are described under the secondary-structure model. (b) Binding affinity of PV-RNAs to TLR3 ECD under different pH conditions.32P-labelled PV-RNAs (cPV1 and PV5) were mixed with varying concentrations of hTLR3 ECD protein and passed through a nitrocellulose filter. After washing, bound radioactivity was measured, and binding activities were calculated as a percentage of input RNA before filtration. The apparent dissociation constant (Kd) values calculated for cPV1 and PV5 were 39±16 and 10±3 nM (pH 5.0), and 31±13 and 7±3 nM (pH 6.0), respectively. (c) HEK293 cells were transfected with an empty vector or expression plasmid for WT TLR3 or each TLR3 mutant (H39A, H39E, H60A, H60E and H539A), together with the IFN-β promoter reporter plasmid and phRL-TK. Twenty-four hours post transfection, cells were stimulated with 10 μg ml−1poly(I:C) or PV5 in FCS-free medium. Luciferase activity was measured 6 h after stimulation. Representative data from three independent experiments are shown. Figure 3: Both N- and C-terminal dsRNA-binding sites of TLR3 are required for PV-RNA-induced TLR3 activation. ( a ) Secondary structure of PV-RNAs (cPV1, PV5 and PV6) predicted by the mfold software. Thick lines indicate dsRNA regions (1–11 bp). The starting and ending positions of ds regions are shown with the nt number. A total number of base pair and the number of nts involved in base pairing in cPV1, PV5 and PV6 are described under the secondary-structure model. ( b ) Binding affinity of PV-RNAs to TLR3 ECD under different pH conditions. 32 P-labelled PV-RNAs (cPV1 and PV5) were mixed with varying concentrations of hTLR3 ECD protein and passed through a nitrocellulose filter. After washing, bound radioactivity was measured, and binding activities were calculated as a percentage of input RNA before filtration. The apparent dissociation constant (Kd) values calculated for cPV1 and PV5 were 39±16 and 10±3 nM (pH 5.0), and 31±13 and 7±3 nM (pH 6.0), respectively. ( c ) HEK293 cells were transfected with an empty vector or expression plasmid for WT TLR3 or each TLR3 mutant (H39A, H39E, H60A, H60E and H539A), together with the IFN-β promoter reporter plasmid and phRL-TK. Twenty-four hours post transfection, cells were stimulated with 10 μg ml −1 poly(I:C) or PV5 in FCS-free medium. Luciferase activity was measured 6 h after stimulation. Representative data from three independent experiments are shown. Full size image We then tested the binding ability of intact PV5 and cPV1 to the recombinant TLR3 ectodomain (ECD) protein under the various pH conditions using a filter binding assay [29] . The ability of PV5 to bind TLR3 was higher than cPV1 at low concentrations of TLR3 ECD in an acidic environment (pH 5.0 and 6.0) ( Fig. 3b ). Even in a neutral pH (7.0), PV5 weakly bound to TLR3 ECD, whereas cPV1 remained unbound ( Fig. 3b ). The binding of PV-RNAs to TLR3 ECD was specific because unlabelled PV5 inhibited the 32 P-labelled PV5 binding dose-dependently. In addition, dsDNA (200 bp in length) hardly bound to TLR3 ECD under any pH condition ( Supplementary Fig. S4 ). TLR3 ECD is composed of 23 leucine-rich repeats (LRRs) and the N- and C-terminal flanking regions [30] . Structural analysis of mouse TLR3 ECD–dsRNA complex revealed that TLR3 ECD dimerized on 46-bp dsRNA [31] . dsRNA interacted with both an N- and C-terminal-binding site on the glycan-free surface of each TLR3 ECD, which are on opposite sides of the dsRNA. The point mutation analyses of human/mouse TLR3 demonstrated that H539 and N541 located in LRR20, H39 in LRR-NT and H60 in LRR1 form the C- and N-terminal-binding site, and are essential for dsRNA-induced TLR3-mediated signalling [29] , [32] . We therefore investigated whether PV5, like dsRNA, activates TLR3 through interaction with the N- and C-terminal-binding sites of TLR3. When TLR3 mutants, in which H39, H60 or H539 was substituted with Ala or Glu, were expressed in HEK293 cells, PV5 failed to induce IFN-β promoter activation, similar to poly(I:C) ( Fig. 3c ). Thus, PV5 appears to interact with the N- and C-terminal dsRNA-binding sites of TLR3 and oligomerize the receptor, leading to the activation of downstream signalling molecules. However, we cannot rule out the possibility that amino acids of the TLR3 ECD, irrelevant to the direct dsRNA binding, participate in the interaction with PV-RNAs. PV5 is internalized and colocalizes with endosomal TLR3 TLR3 activation by poly(I:C) requires clathrin-mediated internalization of extracellular poly(I:C) [33] . In human myeloid DCs and epithelial cells such as HeLa cells, the cytoplasmic raft protein, raftlin, induces poly(I:C) uptake through interaction with clathrin–AP-2 complex [34] , [35] . To understand how extracellular PV-RNAs activate endosomal TLR3, we examined the requirement of raftlin in PV-RNA-induced TLR3 activation by gene silencing of raftlin with small interfering RNA (siRNA). PV-ssRNA or -dsRNA-induced IFN-β promoter activation was greatly decreased when raftlin was knocked down in HEK293 cells, similar to what was observed with poly(I:C) stimulation ( Fig. 4a ). Furthermore, raftlin-knockdown HeLa cells were also impaired in their ability to induce the expression of IFN-β mRNA in response to PV5 ( Fig. 4b ). Again, TICAM-1 was essential for PV-RNA-induced signalling ( Fig. 4a ). 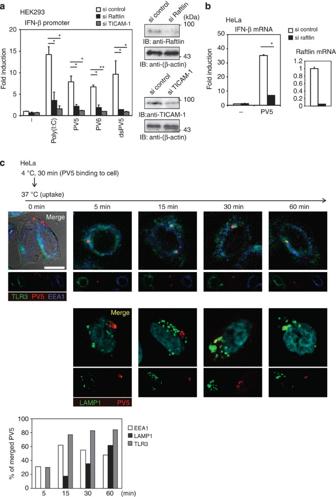Figure 4: Raftlin-mediated endocytosis is essential for PV-RNA-induced IFN-β production by human cells. (a) Left panels: HEK293 cells were transfected with control, raftlin or TICAM-1 siRNAs (20 pmol), together with the expression vector for human TLR3 and the IFN-β reporter plasmid. Forty-eight hours after transfection, cells were washed and stimulated with 20 μg ml−1poly(I:C) or PV-RNAs. After 6 h, luciferase reporter activity was measured and expressed as the fold induction relative to the activity of unstimulated cells. Representative data from three independent experiments are shown (mean±s.d.). Student’st-test was used for statistical analysis. *P<0.05 and **P<0.01. Right panels: Knockdown of raftlin or TICAM-1 was confirmed using western blotting. (b) HeLa cells were transfected with the control or raftlin siRNAs. Forty-eight hours after transfection, cells were washed and stimulated with 20 μg ml−1PV5 for 3 h. Total RNA was extracted, and quantitative PCR was performed using primers for the IFN-β and raftlin genes. Expression of genes was normalized to glyceraldehyde 3-phosphate dehydrogenase mRNA expression. Data are shown as the mean±s.d. Representative data from three independent experiments are shown. *P<0.05. (c) HeLa cells were incubated with 15 μg ml−1Cy3-PV5 for 30 min at 4 °C. After washing, cells were incubated for up to 60 min at 37 °C. At timed intervals, cells were fixed and permeabilized. After staining with anti-TLR3 mAb and anti-EEA1 pAb (upper panels) or anti-LAMP1 mAb (lower panels), cells were incubated with an Alexa Fluor-488- or -633-conjugated secondary Ab and then analysed using confocal microscopy. Red, Cy3-PV5; green, TLR3 or LAMP1; blue, EEA1; light blue, nuclei with 4',6-diamidino-2-phenylindole; white, merged PV5 with TLR3 and EEA1; and yellow, merged PV5 with LAMP1. Scale bar, 10 μm. Co-localization between PV5 and TLR3, EEA1 or LAMP1 was analysed by counting the merged PV5 spots with each molecule in 70 PV5-internalizing cells. The data are shown as % of merged PV5 with EEA1, LAMP1 or TLR3 at indicated time points. Figure 4: Raftlin-mediated endocytosis is essential for PV-RNA-induced IFN-β production by human cells. ( a ) Left panels: HEK293 cells were transfected with control, raftlin or TICAM-1 siRNAs (20 pmol), together with the expression vector for human TLR3 and the IFN-β reporter plasmid. Forty-eight hours after transfection, cells were washed and stimulated with 20 μg ml −1 poly(I:C) or PV-RNAs. After 6 h, luciferase reporter activity was measured and expressed as the fold induction relative to the activity of unstimulated cells. Representative data from three independent experiments are shown (mean±s.d.). Student’s t -test was used for statistical analysis. * P <0.05 and ** P <0.01. Right panels: Knockdown of raftlin or TICAM-1 was confirmed using western blotting. ( b ) HeLa cells were transfected with the control or raftlin siRNAs. Forty-eight hours after transfection, cells were washed and stimulated with 20 μg ml −1 PV5 for 3 h. Total RNA was extracted, and quantitative PCR was performed using primers for the IFN-β and raftlin genes. Expression of genes was normalized to glyceraldehyde 3-phosphate dehydrogenase mRNA expression. Data are shown as the mean±s.d. Representative data from three independent experiments are shown. * P <0.05. ( c ) HeLa cells were incubated with 15 μg ml −1 Cy3-PV5 for 30 min at 4 °C. After washing, cells were incubated for up to 60 min at 37 °C. At timed intervals, cells were fixed and permeabilized. After staining with anti-TLR3 mAb and anti-EEA1 pAb (upper panels) or anti-LAMP1 mAb (lower panels), cells were incubated with an Alexa Fluor-488- or -633-conjugated secondary Ab and then analysed using confocal microscopy. Red, Cy3-PV5; green, TLR3 or LAMP1; blue, EEA1; light blue, nuclei with 4',6-diamidino-2-phenylindole; white, merged PV5 with TLR3 and EEA1; and yellow, merged PV5 with LAMP1. Scale bar, 10 μm. Co-localization between PV5 and TLR3, EEA1 or LAMP1 was analysed by counting the merged PV5 spots with each molecule in 70 PV5-internalizing cells. The data are shown as % of merged PV5 with EEA1, LAMP1 or TLR3 at indicated time points. Full size image Immunofluorescent analyses demonstrated that surface-bound Cy3-labelled PV5 was internalized within a 5-min incubation at 37 °C. PV5 colocalized with TLR3 and the early endosome marker, EEA1, after 15 min, and this was sustained for up to 60 min ( Fig. 4c ). In contrast, co-localization of Cy3-PV5 with LAMP1, a late endosome/lysosome marker, was observed after incubation for 30 min ( Fig. 4c ). The internalization of PV5 was similar to that of poly(I:C) [35] . Indeed, PV5 activity was inhibited by the pre-treatment of cells with B-type CpG oligodeoxynucleotide (ODN), which shares an uptake receptor with poly(I:C) ( Supplementary Fig. S5 ). Taken together, these results strongly suggest that functional PV-RNAs use the poly(I:C)/ODN-uptake receptor for raftlin-mediated endocytosis and that long-term retention of PV5 in the early endosome allows TLR3 to oligomerize for IFN-β production in human cells. PV-RNAs induce TLR3-dependent IFN production by mouse DCs To show the TLR3 dependency in PV-RNA-induced cellular responses, mouse macrophages and DCs from WT or TLR3-deficient mice were used for cytokine assay. When bone marrow-derived macrophages from WT mice were stimulated with cPV1, PV5, PV6 or dsPV5 in the FCS-containing medium, they produced IFN-β in response to PV5, PV6 or dsPV5 ( Supplementary Fig. S6 ). Similarly, splenic CD11c + DCs produced significant amounts of IFN-α/β, TNF-α and IL-6 in response to PV5, PV6 or dsPV5 in the FCS-containing medium ( Fig. 5a ). The activity of PV-RNAs were augmented in FCS-free medium ( Supplementary Fig. S7 ). Unlike human fibroblasts and epithelial cells, mouse CD11c + DCs produced cytokines in response to cPV1 with or without FCS in the media, although the levels were relatively low compared with those induced by exposure to PV5, PV6 or dsPV5. Notably, PV-RNA-induced cytokine production was absent from TLR3-deficient DCs ( Fig. 5a ). Remarkably, cPV1 induced substantial production of proinflmmatory cytokines in FCS-free medium by mouse splenic CD8α + DCs, expressing a high level of TLR3 in a TLR3-dependent manner, similar to cells cultured with PV5, PV6 or dsPV5 ( Supplementary Fig. S8 ). One possible interpretation of these results is that intact cPV1 possesses TLR3-activating ability and that CD11c + or CD8α + DCs promptly take up intact cPV1 before being degraded in FCS-free or -containing medium and deliver it to the endosomal compartment where TLR3 resides. Indeed, intact cPV1 bound to the TLR3 ECD under acidic conditions, though with lower affinity than PV5 ( Fig. 3b ). When PV5 was pre-treated with RNaseIII, a dsRNA-specific RNase, cytokine production by splenic CD11c + DCs was abrogated, indicating that RNA duplex is required for PV5-induced TLR3 activation ( Fig. 5b ). 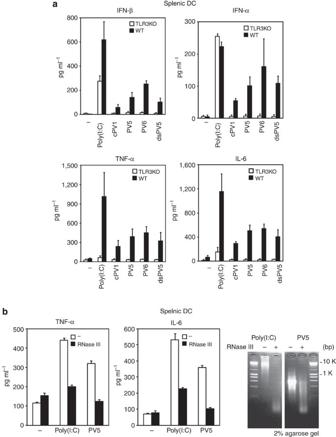Figure 5: Mouse splenic DCs produce type I IFN and cytokines in response to PV-RNAs in a TLR3-dependent manner. (a) Splenic CD11c+DCs (1 × 106per ml) isolated from TLR3−/−or WT mice were stimulated with 20 μg ml−1poly(I:C) or PV-derived RNAs in FCS-containing medium. Twenty-four hours after stimulation, culture supernatants were collected, and IFN-α/β in the supernatants was quantified using ELISA. TNF-α and IL-6 levels were measured using CBA. Representative data from three independent experiments are shown (mean±s.d.). (b) Poly(I:C) and PV5 (20 μg ml−1) were pre-treated with RNaseIII for 30 min at 37 °C or left untreated before adding to CD11+splenic DCs (1 × 106per ml) isolated from WT mice. Twenty-four hours after stimulation, TNF-α and IL-6 levels were measured in culture supernatants using CBA (left panels). RNaseIII-treated poly(I:C) and PV5 were electrophoresed on a 2% agarose gel (right panels). Figure 5: Mouse splenic DCs produce type I IFN and cytokines in response to PV-RNAs in a TLR3-dependent manner. ( a ) Splenic CD11c + DCs (1 × 10 6 per ml) isolated from TLR3 −/− or WT mice were stimulated with 20 μg ml −1 poly(I:C) or PV-derived RNAs in FCS-containing medium. Twenty-four hours after stimulation, culture supernatants were collected, and IFN-α/β in the supernatants was quantified using ELISA. TNF-α and IL-6 levels were measured using CBA. Representative data from three independent experiments are shown (mean±s.d.). ( b ) Poly(I:C) and PV5 (20 μg ml −1 ) were pre-treated with RNaseIII for 30 min at 37 °C or left untreated before adding to CD11 + splenic DCs (1 × 10 6 per ml) isolated from WT mice. Twenty-four hours after stimulation, TNF-α and IL-6 levels were measured in culture supernatants using CBA (left panels). RNaseIII-treated poly(I:C) and PV5 were electrophoresed on a 2% agarose gel (right panels). Full size image The estimated secondary-structure model of PV5 To clarify the secondary structure of PV5, we performed the partial digestion of PV5 using MazF at room temperature. MazF is an ACA-specific endoribonuclease that specifically cleaves ssRNA regions at the 5′-end of the ACA sequence, but not dsRNA regions [36] . Cleavage occurs at the 5′ end of the first A residue in an ACA sequence, which produces 2′,3′-cyclic phosphate and the other 5′ OH group [37] . There are 12 ACA sites in PV5. Therefore, to estimate the size of cleaved fragments, PV5-deletion mutants were also digested with MazF ( Fig. 6a ). Comparison of the cleaved fragments with the mutant RNAs clearly demonstrated that the 124 ACA site in PV5, which was expected to be a dsRNA region, was resistant to cleavage ( Fig. 6b ). At approximately the 40-mer RNA position, two fragments were detected in PV5(456)/MazF and PV5/MazF. The slow-migration band intensity increased in a time-dependent manner and the fast-migration band intensity gradually decreased. This indicated that the former may be the final digested fragment and the latter was at an intermediate stage of digestion. This was confirmed by additional digestion analyses ( Supplementary Fig. S9 ). We compared our data with several secondary-structure models (RNAfold, mfold and centroidfold) of PV5 and determined that the mfold secondary-structure model was most fitted among them ( Fig. 6b and Supplementary Fig. S10 ). 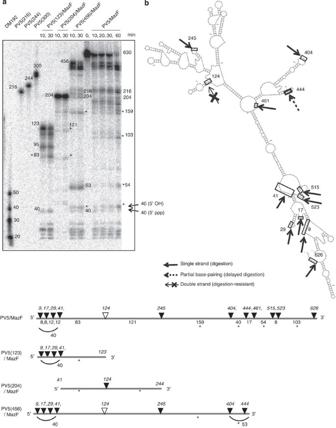Figure 6: Partial digestion of PV5 with MazF. (a) MazF-induced cleavage pattern of PV5 and the deletion mutants visualized on a denaturing 5% PAGE. PV5 was digested with MazF at room temperature, and other RNAs were digested at 37 °C. The cleavage pattern is schematically drawn at the bottom of the figure. MazF recognized ACA-cleavage sites are indicated by triangles. Black triangles indicate the observed cleavage sites and white triangles indicate sites not detected on the gel. Asterisks indicate the fragments produced by MazF-mediated ACA-specific digestion. Italic letters show the position numbers of the first A residues in ACA sequences of PV5. RNA size markers: DM192 (20-, 30-, 40- or 50-mer, Bio Dynamics Laboratory Inc.), PV5(216)(216-mer), PV5(244)(244-mer) and PV5(300)(300-mer). (b) Secondary structure of PV5 predicted by the mfold software. Rectangles show the ACA sites of PV5. The position numbers of the first A residues in ACA sequences of PV5 are shown. Solid arrows indicate the MazF-digestion sites. Broken arrow indicates the delayed digestion site. Figure 6: Partial digestion of PV5 with MazF. ( a ) MazF-induced cleavage pattern of PV5 and the deletion mutants visualized on a denaturing 5% PAGE. PV5 was digested with MazF at room temperature, and other RNAs were digested at 37 °C. The cleavage pattern is schematically drawn at the bottom of the figure. MazF recognized ACA-cleavage sites are indicated by triangles. Black triangles indicate the observed cleavage sites and white triangles indicate sites not detected on the gel. Asterisks indicate the fragments produced by MazF-mediated ACA-specific digestion. Italic letters show the position numbers of the first A residues in ACA sequences of PV5. RNA size markers: DM192 (20-, 30-, 40- or 50-mer, Bio Dynamics Laboratory Inc.), PV5(216)(216-mer), PV5(244)(244-mer) and PV5(300)(300-mer). ( b ) Secondary structure of PV5 predicted by the mfold software. Rectangles show the ACA sites of PV5. The position numbers of the first A residues in ACA sequences of PV5 are shown. Solid arrows indicate the MazF-digestion sites. Broken arrow indicates the delayed digestion site. Full size image The core RNA structure required for TLR3 activation Based on the mfold model, we attempted to identify the core RNA structure required for TLR3 activation in PV5. PV5-derived RNAs partly having PV5 secondary structure (PV5-D1–PV5-D5) were made by in vitro transcription ( Fig. 7a ), and their stability and TLR3-activating ability were assessed. PV5-D1, D3 and D5 were resistant to degradation, and extracellularly activate TLR3 similar to PV5, leading to IFN-β promoter activation in HEK293 cells and cytokine production in mouse splenic DCs or bone marrow-derived macrophages ( Fig. 7b–d ). In contrast, PV5-D2 and -D4, which were resistant to degradation in FCS-free medium but were readily degraded in FCS-containing medium, failed to induce TLR3-mediated IFN-β promoter activation by either extracellular stimulation in FCS-free medium or direct endosomal delivery using DOTAP ( Fig. 7b ). When PV5-D2 and -D4 were added to mouse splenic DCs or bone marrow-derived macrophages in the FCS-free conditions, IFN-β and proinflammatory cytokines, including TNF-α and IL-6, were produced in a TLR3-dependent manner, though their levels were relatively low compared with those induced by PV5-D1, D3 or D5 ( Fig. 7d ). These results suggest that longer stem structure with bulge and internal loops typically shown in PV5-D5 mfold model is the core RNA structure required for TLR3 activation in PV5 and also in PV6. In addition, shorter mismatched RNA duplexes such as PV5-D2 and -D4 can be recognized by TLR3 with less activity in mouse DCs/macrophages if they hold the structure, which differs from TLR3 response in HEK293 cells. Given that RNA molecules have an appropriate tertiary interactions, the stability and TLR3-binding ability of these RNA molecules must be influenced by RNA tertiary structure. 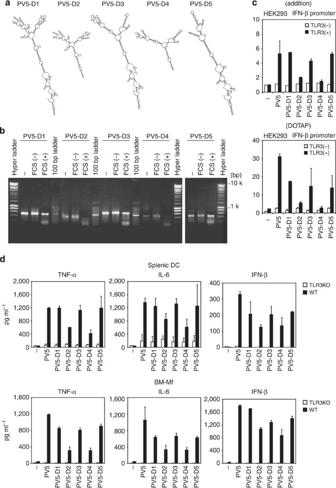Figure 7: Mapping of TLR3-activating RNA structure in PV5. (a) Secondary structure of PV5-derived RNAs (PV5-D1–PV5-D5) predicted by the mfold software. (b) RNAs were incubated in FCS-free or -containing medium at 37 °C. Non-treated RNA or RNA incubated for 30 min were loaded onto a 1% agarose gel. (c) TLR3-mediated IFN-β promoter activation induced by PV5 or PV5-derived RNAs in HEK293 cells transiently expressing TLR3. Cells were stimulated with indicated RNAs (10 μg ml−1) (upper panel) or RNAs complexed with DOTAP (1 μg ml−1) (lower panel). After 6 h, luciferase reporter activity was measured and expressed as the fold induction relative to the activity of unstimulated cells. Data are shown as the mean±s.d. Representative data from three independent experiments are shown. (d) Splenic CD11c+DCs (upper panels) or bone marrow-derived macrophages (lower panels) (2 × 106per ml) isolated from TLR3−/−or WT mice were stimulated with 100 pmol ml−1PV5 or PV5-derived RNAs in FCS-free AIM medium. Twenty-four hours after stimulation, culture supernatants were collected, and IFN-β in the supernatants was quantified using ELISA. TNF-α and IL-6 levels were measured using CBA. Representative data from three independent experiments are shown (mean±s.d.). Figure 7: Mapping of TLR3-activating RNA structure in PV5. ( a ) Secondary structure of PV5-derived RNAs (PV5-D1–PV5-D5) predicted by the mfold software. ( b ) RNAs were incubated in FCS-free or -containing medium at 37 °C. Non-treated RNA or RNA incubated for 30 min were loaded onto a 1% agarose gel. ( c ) TLR3-mediated IFN-β promoter activation induced by PV5 or PV5-derived RNAs in HEK293 cells transiently expressing TLR3. Cells were stimulated with indicated RNAs (10 μg ml −1 ) (upper panel) or RNAs complexed with DOTAP (1 μg ml −1 ) (lower panel). After 6 h, luciferase reporter activity was measured and expressed as the fold induction relative to the activity of unstimulated cells. Data are shown as the mean±s.d. Representative data from three independent experiments are shown. ( d ) Splenic CD11c + DCs (upper panels) or bone marrow-derived macrophages (lower panels) (2 × 10 6 per ml) isolated from TLR3 −/− or WT mice were stimulated with 100 pmol ml −1 PV5 or PV5-derived RNAs in FCS-free AIM medium. Twenty-four hours after stimulation, culture supernatants were collected, and IFN-β in the supernatants was quantified using ELISA. TNF-α and IL-6 levels were measured using CBA. Representative data from three independent experiments are shown (mean±s.d.). Full size image In the current study, we demonstrated, for the first time, that mouse/human TLR3 detects extracellular virus-derived RNA with stable stem structures to induce innate immune signalling. Functional PV-RNAs were degradation-resistant, and their ability to activate TLR3 was dependent on the dsRNA region within the RNA molecule, which is required for interaction with the N- and C-terminal dsRNA-binding sites of the TLR3 ECD. Based on the structural analysis of the TLR3–dsRNA complex, it has been proposed that 40–50 bp dsRNA was the minimum signalling unit with two TLR3 molecules [31] . Jelinek et al . [11] reported that dsRNAs, >90 bp in length, triggered TLR3 oligomerization and efficiently induced IFN-β and TNF-α production in conventional murine DCs. Functional PV-RNAs, such as PV5 and PV6, induced TLR3-dependent IFN-α/β and proinflammatory cytokines from mouse CD11c + DCs ( Fig. 5 ); these RNAs appeared to oligomerize TLR3 molecules even though they harbour bulges and internal loops in their duplex structures. If this is the case, TLR3 recognizes not only perfect duplex of ~90 bp dsRNA but also the mismatched RNA duplex whithin ~600-nt PV-RNA. We identified the core RNA structure required for TLR3 activation in PV5, which is relatively long stem structure with bulge and internal loops typically shown in PV5-D5 mfold secondary structure. The fascinated model for TLR3 dimer formation has been proposed, in which shorter RNA duplexes of between 21 and 30 bp can form less stable complexes with two TLR3 molecules [32] . Thus, TLR3 appears to have flexibility to recognize RNA molecules. Interestingly, PV5 segments (approximately 200 nts in length; PV5 a, b and c) lost the ability to activate TLR3 in HEK293 cells despite their degradation-resistant structure ( Supplementary Fig. S3c ), suggesting that an appropriate topology of multiple RNA duplexes are required for TLR3 activation. In addition, PV5-D2 and -D4 failed to activate IFN-β promoter in HEK293 cells expressing TLR3, but efficiently induced type I IFN and proinflammatory cytokine production from mouse splenic DCs and bone marrow-derived macrophages in a TLR3-dependent manner ( Fig. 7 ). Recently, it has been reported that TLR3 undergoes cathepsin-mediated proteolytic processing, and both full-length and C-terminal cleaved form of TLR3 molecules reside in human retinal epithelial cell line and monocyte-derived DCs [38] . It is interesting if shorter RNAs with mismatched duplex, such as PV5-D2 and -D4, are recognized by protease-processed TLR3 in mouse DCs or bone marrow-derived macrophages with different binding modes from intact TLR3 [38] . Indeed, the cleaved form of TLR3 is predominant in mouse macrophages [39] , but less present in HEK293 cells [40] , which may explain the different TLR3 responses to these RNAs between mouse DCs/macrophages and human HEK293 cells ( Fig. 7 ). There have been many reports indicating that TLR3-dependent inflammatory cytokine and chemokine production affects virus-induced pathology and host survival in RNA virus infections such as respiratory syncytial virus, influenza A virus and phlebovirus, a negative-strand RNA virus that produces minimal dsRNA as an intermediate product [8] . Furthermore, TLR3 functions as an endogenous sensor of necrosis and is required for chemokine production by peritoneal macrophages after co-culture with necrotic neutrophils [24] . However, these biological studies have suffered from the lack of information about the actual molecules sensed by TLR3 in such infection/inflammatory states. More recently, Bernard et al . [41] demonstrated that UV-damaged self-noncoding RNA is detected by TLR3. We suppose that viral/host RNAs with stable stem structures derived from infection- or inflammation-damaged cells activate TLR3 to induce cytokine and chemokine production. In the case of PV infection, TLR3-mediated type I IFN production is important for viral clearance in vivo [15] , [16] . In vitro PV infection of splenic DCs promotes type I IFN production in a TLR3-dependent manner. The positive-stranded ssRNAs and the replicative form are robustly present in PV-infected cells, which might be segmented into functional ssRNAs similar to PV5 and PV6 extracellularly due to necrosis. Hence, in the local environment, segmented virus-derived structured RNAs can function as a TLR3 ligand. The flexible RNA-recognition mode of TLR3 may have some advantage to protect host against wide spectrum of virus infection. Notably, RNA uptake is required for TLR3 signalling. Functional PV-RNAs possess the essential structural elements required for both cellular uptake and TLR3 oligomerization. We found that raftlin, a cytoplasmic lipid raft protein, is a molecule that participates in uptake of PV-RNAs and delivery to TLR3-positive early endosomes ( Fig. 4 ). The features of the TLR3-recognizing PV-RNAs are consistent with our previous results that raftlin mediates poly(I:C) cellular uptake through interaction with the clathrin–AP-2 complex in human myeloid DCs and epithelial cells [35] . In addition, uptake of B/C-type CpG ODNs that share their uptake receptor with poly(I:C) was also mediated by raftlin [33] , [35] . Given that PV5-induced TLR3 activation in HEK293 cells was inhibited by pre-treatment with the B-type CpG ODN ( Supplementary Fig. S5 ), PV5 likely utilizes the poly(I:C)/ODN-uptake receptor for endocytosis. Although CD14 and the scavenger receptor class A were reported to act as a poly(I:C)-uptake receptor in mouse macrophages and human bronchial epithelial cells, respectively [42] , [43] , they did not participate in poly(I:C)/ODN cellular uptake in human DCs because of their absence on the cell surface [12] . There must be an additional uptake receptor for poly(I:C)/ODN. Identification of the uptake receptor for virus RNAs is important for improving our understanding of the innate immune response to viral infection and sterile inflammation. TLRs recognize pathogen- or damage-associated molecular patterns and promote the activation of the innate and adaptive immune responses through ligand-induced oligomerization [44] , [45] . Structural analyses of TLR3, TLR4, TLR5, TLR2/1 and TLR2/6 ECDs, and their complexes with typical ligands, demonstrated that each TLR possessed ligand-binding sites or pockets and a dimerizing interface, which allowed for ligand-induced receptor dimerization [46] , [47] . Although there are multiple ligands for each TLR, it remains unknown whether they share common structural features. The current study is the first to characterize the RNA structure capable of triggering TLR3 activation and demonstrate that viral RNAs with intermittent stem structure are recognized by an uptake receptor and by TLR3, inducing innate immune signalling. Precise analyses of the mechanisms underlying pattern recognition by TLRs using different ligands might be important for engineering synthetic TLR-activating ligands. Cell culture and reagents HEK293 and Vero cells were maintained in DMEM (Invitrogen) supplemented with 10% heat-inactivated FCS (Invitrogen) and antibiotics. HeLa cells were kindly provided by Dr T. Fujita (Kyoto University) and maintained in Eagle’s minimal essential medium (Nissui, Tokyo, Japan) supplemented with 1% L -glutamine and 5% heat-inactivated FCS. Normal embryonic lung fibroblasts, MRC5 cells, were maintained in MEM-alpha (Invitrogen) supplemented with 10% heat-inactivated FCS and antibiotics. The anti-human TLR3 monoclonal antibody (mAb) (clone TLR3.7) was generated in our laboratory [5] . The anti-human raftlin polyclonal Ab (pAb) and anti-mouse TLR3 mAb were kindly provided by Dr K. Saeki (Kyushu University) and Dr D. M. Segal (National Institutes of Health, MD), respectively. [34] , [11] Anti-EEA1 pAb (PA1-063) was purchased from Affinity Bioreagents; anti-β-actin mAb (A2228) was purchased from Sigma; the anti-LAMP1 mAb (328601) was purchased from Biolegend; the anti-TICAM-1 pAb (4596) was purchased from Cell Signaling; and Alexa Fluor-488 and -633-conjugated secondary antibodies were purchased from Invitrogen. Poly(I:C) was purchased from Amersham Biosciences. RNase A and RNase III were purchased from Ambion. Mice Inbred C57BL/6 WT mice were purchased from CLEA Japan (Tokyo, Japan). TLR3 −/− mice were provided by Dr S. Akira (Osaka University). Mice were maintained under specific pathogen-free conditions in the animal facility of the Hokkaido University Graduate School of Medicine. Female mice of 6–10 week of age were used in all experiments that were performed according to the guidelines established by the Hokkaido University Animal Care and Use Committee. Plasmids The cDNA fragments encoding the open-reading frame of human TLR3 was amplified using RT–PCR with total RNA prepared from monocyte-derived DCs and was ligated into the cloning site of the expression vector, pEF-BOS, which was a gift from Dr S. Nagata (Kyoto University) [48] . Mahoney PV complementary DNA was provided by Dr S. Koike (Tokyo Metropolitan Institute of Medical Science, Tokyo). TLR3-mutant plasmids were gifts from Dr K. Fukuda (Yamagata University) [29] . RNA extraction from PV-infected cells Vero cells were infected with PV or not infected. Forty-eight hours later, cells and culture supernatants were divided by centrifugation (2,000 r.p.m., 10 min). TRIzol reagent (Invivogen) was added to cell pellets for extraction of RNA. Obtained RNAs were purified by ethanol precipitation, and concentration was determined by measuring the absorbance at 260 nm in a spectrophotometer. Preparation of RNA DNA fragments containing the PV gene segment and the T7 promoter sequence were amplified using PCR with specific primers and the PV-cDNA as a template ( Supplementary Table S2 ). The PV sense and antisense RNAs from the PCR products were transcribed in vitro using an AmpliScribe T7 transcription kit (Epicentre Technologies, Madison, WI, USA) according to the manufacturer’s protocol. The transcribed products were separated on a 1% agarose gel, and the band corresponding to PV RNA was excised using RECOCHIP (Takara). Then, eluted RNAs were ethanol precipitated and resuspended in RNase-free water. To generate dsRNA, sense and antisense RNAs were annealed. PV-ss/dsRNAs were pre-treated with polymyxin B (5 μg ml −1 ) for 1 h before being added to mouse macrophages and DCs. RNA was labelled with Cy3 maleimide mono-reactive dye (GE Healthcare) using the 5′ EndTag Nucleic Acid Labeling System (Vector Laboratories, Inc.). Cy3-PV5 showed a full activity. Reporter gene assay HEK293 cells (8 × 10 5 cells per well) were cultured in six-well plates and transfected with the TLR3-expression vector or an empty vector (400 ng per well), together with the reporter plasmid (400 ng per well) and an internal control vector phRL-TK (Promega, Madison, WI, USA) (20 ng per well) using FuGENE HD (Roche). The p-125 luc reporter containing the human IFN-β promoter region (−125 to +19) was provided by Dr T. Taniguchi (University of Tokyo). After 24 h, cells were collected and resusupended with FCS-free or -containing medium. Then, cells were seeded on 96-well plates and stimulated with the indicated RNAs. Six hours later, cells were lysed using the passive lysis buffer (Promega), and Firefly and Renilla luciferase activities were determined using a dual-luciferase reporter assay kit (Promega). The Firefly luciferase activity was normalized by Renilla luciferase activity and was expressed as the fold stimulation relative to activity in non-stimulated cells. Filter binding assay Radioisotope labelling of PV-RNAs by in vitro transcription with [α- 32 P-ATP] was carried out as previously decribed [49] . Labelled PV-RNAs (2 nM) were mixed with varying concentrations (none or 6.25, 12.5 25, 50, 100 or 200 nM) of human TLR3 (amino acid 27–711; R&D Systems) and adjusted to a total volume of 25 μl using binding buffer (pH 5.0–7.0) containing 100 mM NaCl (20 mM AcONa (pH 5.0–6.0) or 20 mM Tris–HCl (pH 6.5–7.0)). After 30 min incubation, the mixtures were passed through a nitrocellulose filter and washed twice with 500 μl reaction buffer. The amount of bound RNA was measured using BAS 2500 (Fujifilm), and binding activities were calculated as the percentage of input RNA. Quantitative PCR Total RNA was extracted using the RNeasy mini kit (Qiagen, Valencia, CA) and reverse transcribed using the High Capacity cDNA Reverse Transcripition kit (Applied Biosystems) and random primers according to the manufacturer’s instructions. qPCR was performed using the indicated primers ( Supplementary Table S3 ) and the Step One Real-time PCR system (Applied Biosystems). RNA interference and immunoblotting siRNA duplexes (Raftlin, catalogue number s23219; negative control, catalogue number AM4635) were purchased from Ambion-Applied Biosystems. siRNA for TICAM-1 was purchased from Xeragon Inc. (Birmingham, AL, USA). HEK293 cells were cultured in 24-well plates and transfected with 20 pmol each siRNA, together with the expression vector for human TLR3 (200 ng), IFN-β promoter plasmid (100 ng) and an internal control vector (1.5 ng) using Lipofectamine 2000. Forty-eight hours after transfection, cells were stimulated with 10 μg ml −1 ligands for 6 h. Cells were lysed and dual-luciferase activities were measured according to the manufacturer’s instructions (Promega). Cell lysates were clarified by centrifugation and mixed with denaturing buffer. Samples were analysed using 10% SDS–PAGE followed by immunoblotting with anti-raftlin pAb (1/1,000), anti-β-actin mAb (1/1,000) or anti-TICAM-1 pAb (1/500). In the case of HeLa cells, cells cultured in 12-well plates were transfected with 40 pmol each siRNA using Lipofectamine 2000. Confocal microscopy HeLa cells (1.0 × 10 5 cells per well) were plated onto micro-cover glasses (Matsunami, Tokyo, Japan) in a 12-well plate. The following day, cells were incubated with 15 μg ml −1 Cy3-labelled PV5 for 30 min at 4 °C. Cells were washed twice and further incubated for 5–60 min at 37 °C. At timed intervals, cells were fixed with 4% paraformaldehyde for 15 min and permeabilized using PBS containing 0.2% Triton and 1% BSA for 15 min. Fixed cells were labelled with anti-EEA1 pAb (1/200), anti-LAMP1 mAb (1/300) or anti-human TLR3 mAb (1/50) overnight at 4 °C. Then, Alexa Fluor-488- or -633-conjugated secondary Abs (1/400) were used to visualize the primary Abs. Prolong Gold was used for staining the nuclei. Cells were visualized at a × 63 magnification using an LSM510 META microscope (Zeiss, Jena, Germany). Purification of mouse DCs from spleen Splenocytes from WT or TLR3 −/− mice were treated with 400 IU MandleU per ml collagenase D (Roche) at 37 °C for 25 min in HBSS (Sigma-Aldrich). EDTA was added to the cell suspensions and incubated for an additional 5 min at 37 °C. After lysis of red blood cells using the ACK lysis buffer, splenocytes were incubated with magnetic-activated cell sorting anti-CD11c-conjugated microbeads, and DCs were purified using magnetic separation columns as indicated by the manufacturer (Miltenyi Biotec, Auburn, CA, USA). Positively selected cells were isolated and suspended in RPMI 1640 (Invitrogen) supplemented with 10% heat-inactivated FCS and antibiotics. For isolation of CD8α + DCs, the magnetic-activated cell sorting CD8α + DC-positive selection kit was used according to the manufacturer's instructions. Purity was checked routinely by FACS and was found to be >80% (CD11c + ) or >90% (CD8α + ), respectively. Enzyme-linked immunosorbent assay and cytometric bead array Cells were stimulated with the indicated RNAs in FCS-containing medium or FCS-free AIM-V medium (Invitrogen). Twenty-four hours after stimulation, culture supernatants were collected and analysed for cytokine levels with enzyme-linked immunosorbent assay (ELISA) or cytometric bead array (CBA). ELISA kits for IFN-α and IFN-β were purchased from PBL Biomedical Laboratories and were performed according to the manufacturer’s instructions. CBA flex sets for mouse IL-6 and TNF-α were purchased from BD Bioscience. Experiments were performed according to the manufacturer’s instructions, and samples were analysed using the FacsAria (BD Bioscience). Statistical analysis Statistical significance of differences between groups was determined by the Student’s t -test. Prediction of RNA secondary structure The secondary structure of RNAs was modelled using mfold ( http://mfold.rna.albany.edu/?q.mfold ), RNAfold ( http://rna.tbi.univie.ac.at/cgi-bin/RNAfold.cgi ) and centroidfold program ( http://www.ncrna.org/software/centroidfold/ ). How to cite this article: Tatematsu, M. et al . Toll-like receptor 3 recognizes incomplete stem structures in single-stranded viral RNA. Nat. Commun. 4:1833 doi: 10.1038/ncomms2857 (2013).